Social networks reveal cultural behaviour in tool-using dolphins Animal tool use is of inherent interest given its relationship to intelligence, innovation and cultural behaviour. Here we investigate whether Shark Bay bottlenose dolphins that use marine sponges as hunting tools (spongers) are culturally distinct from other dolphins in the population based on the criteria that sponging is both socially learned and distinguishes between groups. We use social network analysis to determine social preferences among 36 spongers and 69 non-spongers sampled over a 22-year period while controlling for location, sex and matrilineal relatedness. Homophily (the tendency to associate with similar others) based on tool-using status was evident in every analysis, although maternal kinship, sex and location also contributed to social preference. Female spongers were more cliquish and preferentially associated with other spongers over non-spongers. Like humans who preferentially associate with others who share their subculture, tool-using dolphins prefer others like themselves, strongly suggesting that sponge tool-use is a cultural behaviour. For centuries, philosophers and scientists have debated whether cultural behaviour distinguishes Homo from all other taxa [1] , [2] . Whether non-human animals have at least rudimentary culture is contested, partly because scholars disagree on the definition of culture and/or what type of supporting evidence is needed [2] . To empirically investigate whether or not a given species has 'culture,' the term must be operationally defined. Regardless of discipline, scholars agree that some form of social learning is a prerequisite and that culture is a source of uniformity within groups and differences between groups [3] , but the consensus ends here. Social learning is defined as learning (behaviour matching) that is influenced by observation of, or interaction with another animal or its products [4] , [5] . Some definitions of culture require more complex cognitive social learning mechanisms, such as pedagogy, theory of mind and imitation [6] , [7] . In most animal culture studies, examination of behavioural variation within and between groups is fairly straightforward as animals are either geographically or socially segregated [2] . However, 'group' is not easily defined in all animal societies. Like humans, Shark Bay bottlenose dolphins live in an open community, characterized by high fission–fusion dynamics where members maintain long-term preferential bonds, but associations are temporally and spatially variable across minutes, days and years [8] . The question is therefore whether dolphins that use sponge tools (spongers) to extract prey [9] , [10] exhibit homophily (the tendency to associate with similar others), based on this socially learned foraging tactic [10] , [11] . In Shark Bay, Australia, a subset of the community of Indo-Pacific bottlenose dolphins ( Tursiops sp.) procure and wear basket sponges on their beaks while lightly scouring the seafloor for prey in deep (8–13 m) channels ( Fig. 1 ) [9] , [10] , [11] , [12] . Sponging is the best-documented case of tool use by wild cetaceans and is unique among wildlife in that only a small subset of the population uses tools. This exceptional case of tool-use heterogeneity allows us to test for preferential affiliation based on tool-use. To date, 55 dolphins have been documented habitually using sponges in the eastern gulf of Shark Bay [12] , although sponging also occurs in the western gulf [13] . Only calves of spongers become spongers (24 offspring to date), but 8 offspring of spongers never adopted sponging. Sponging is a solitary activity, but calves accompany their mothers during sponging and vertical social learning is strongly implicated as the primary mechanism of transmission [10] , [11] , [14] , consistent with mitochondrial DNA analysis [13] , [15] . 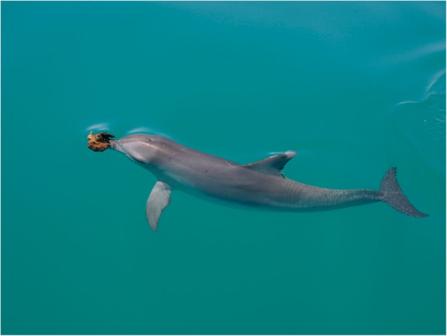Figure 1: Juvenile female sponger. Photo by Ewa Krzyszczyk;http://www.monkeymiadolphins.org. Figure 1: Juvenile female sponger. Photo by Ewa Krzyszczyk; http://www.monkeymiadolphins.org . Full size image The initial 'culture' claim for sponging proved contentious [16] , [17] , [18] , largely stemming from application of the exclusion method [15] to demonstrate social learning, and hence cultural behaviour. This method involves trying to eliminate genetic and environmental explanations for a behavioural variant in a wild population, thus leaving social learning as the most plausible explanation for the variant [19] . The main critique of the exclusion method is that it tries to prove the null and produces false negatives because ecological factors often contribute to cultural behaviour [16] , [20] . Regardless, this method is not appropriate for identifying sponge tool-use as cultural behaviour, as environmental factors cannot be excluded; the deep channels where sponging occurs have high basket sponge density [21] and prey that are difficult to detect without sponge tools [12] . Many, but not all, animals that use these channels specialize in sponging and spongers spend more time using tools than any non-human animal [10] . So, although Krützen et al . [15] did not demonstrate social learning per se , the social contribution is well-documented elsewhere [10] , [11] , [14] and the strong ecological component does not refute the argument that sponging is socially learned. What is lacking, however, is evidence that sponging distinguishes between groups. In virtually all other cases of animal tool-use or a putative cultural behaviour, all members of the group participate. As spongers are a small subset of the community, we can explicitly test for an affiliative function for the behaviour. In other taxa, individuals develop the behaviour because they are part of the group; they do not group because of the behaviour. Unlike tool-users in any other animal population, spongers interact with non-tool users for variable amounts of time. If sponging is a cultural behaviour, it may foster increased affiliation and homogeneity between spongers. This increase in similarity is a natural precursor to conceptions of human culture, which focus on group identity, convention, homophily and adherence to norms [2] , [22] , [23] , [24] . Similar to human subcultures, the dynamic nature of dolphin society allows them to associate based on socially learned behaviours rather than simply conform to the norms of the larger group they happen to be in. Therefore, we are specifically interested in whether foraging similarity is a factor in social preference. As sponging is a solitary behaviour [10] , affiliation between spongers would not be based on collective foraging, but rather on identifying other individuals as spongers. This attraction has adaptive implications, in which homophily is likely to reinforce the socially learned behaviour and influence horizontal information transfer (for example, where to find sponges), even if the behaviour was initially vertically learned from only one parent. We refer to our hypothesis, that spongers preferentially affiliate with other spongers as the 'homophily hypothesis.' In Shark Bay, bottlenose dolphin females form relatively loose kin-based networks [25] , [26] , males form tight long-term alliances, and there is no evidence of emigration [27] . Diverse foraging tactics characterize the population [14] and most are female biased [10] , [28] . Males tend to adopt foraging tactics that are widely used in the population and females are more likely to specialize in tactics that are habitat specific. We attribute the sex difference to the divergent reproductive tactics of males and females. Females require substantial resources to support large dependent offspring that nurse for 3–8 years [29] , and specialization may enable them to meet those energetic demands. Males cannot afford to compromise their fitness by specializing in foraging tactics that would restrict their ability to form and maintain alliances, or range widely to find females. To date, at least three attributes, matrilineal kinship, sex and geographic proximity, influence dolphin association [25] , [26] , [30] , [31] , but affiliation based on foraging type has never been tested. Here we examine social patterns of both female and male spongers and non-spongers. Because sponging does not occur throughout our study area, we control for ecological context by restricting our sample to dolphins with extensive geographic overlap with spongers (see Methods, Fig. 2 ). Within this sample, we examine homophily based on foraging type while statistically controlling for kinship, sex and geographic proximity using the Multiple Regression Quadratic Assignment Procedure (MRQAP [32] ). This permutation method allows us to include multiple matrices in one analysis while accounting for structural autocorrelation that is inherent to social networks as well as discriminate between the multiple factors that are likely to influence association. We found strong support for the homophily hypothesis, suggesting that dolphins form cultural subgroups based on socially learned traits such as sponge tool-use. 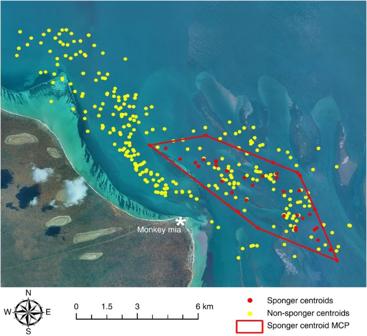Figure 2: Sponger core area. Map of study area and dolphin centroids. Monkey Mia is our boat-launching site. The MCP area outlined in red (22 km2) encompasses centroids for all spongers and contains 105 dolphins. Dolphin home ranges are typically at least twice the size of the core area27, which allows us to ensure considerable overlap between spongers and non-spongers in the Sponger centroids are red; non-sponger centroids are yellow. Figure 2: Sponger core area. Map of study area and dolphin centroids. Monkey Mia is our boat-launching site. The MCP area outlined in red (22 km 2 ) encompasses centroids for all spongers and contains 105 dolphins. Dolphin home ranges are typically at least twice the size of the core area [27] , which allows us to ensure considerable overlap between spongers and non-spongers in the Sponger centroids are red; non-sponger centroids are yellow. Full size image Sex differences in overall social network metrics Using all individuals in our main study area with >11 sightings ( n =421), we examined sex differences for five basic social network metrics ( Table 1 ). As expected, based on male alliance structure [8] , [25] , [31] , permutation tests revealed that males had higher strength, eigenvector centrality and clustering coefficient than females. Given these robust sex differences and the sex difference in sponging, we separated males and females for some subsequent analyses. Table 1 Sex differences in social network metrics. Full size table Social network metrics of female spongers and non-spongers As expected, for animals within the core sponger area ( Fig. 2 , n =105), non-spongers had higher degree, strength and eigenvector centrality than spongers. However, spongers had a higher clustering coefficient than non-spongers, suggesting they were significantly more cliquish ( Table 2 ). Table 2 Social network comparison of female spongers and non-spongers in core area. Full size table Within-group and between-group affinity To explore the relationship between spongers and non-spongers, we compared social affinity indices within and between groups (homophily versus heterophily) for animals located within the core sponger area ( Fig. 2 ). Association within each group (sponger–sponger and non-sponger–non-sponger) was significantly higher (mean±s.e. social affinity index 0.039±0.018) than between groups (sponger–non-sponger) (0.022±0.014; Mantel test, t =7.1433, P <0.0001). The average social affinity index for sponger–sponger associations was 0.030±0.012 and for non-sponger–non-sponger associations was 0.043±0.019. In addition, spongers had a greater proportion of sponger associates (average 0.392±0.021) than non-spongers did (0.278±0.010; Mantel test, t =5.75; P <0.0001; n =105). Sociability based on sex and foraging type In a previous study we found that female spongers were more solitary than non-sponger females [10] , but here we included eight male spongers and males differ from females in terms of sociability in general ( Table 1 ). Consequently, we examined the effects of sex and foraging type on sociability by calculating the proportion of surveys that dolphins were alone (dependent calves excluded) or with at least one other dolphin. A generalized linear mixed model, including the fixed effects sex, foraging type, and the sex by foraging type interaction as well as individual as a random effect, fit the data better than the null model including only the random effect (likelihood ratio test, χ 2 =56.08, d.f.=5, P <0.0001). 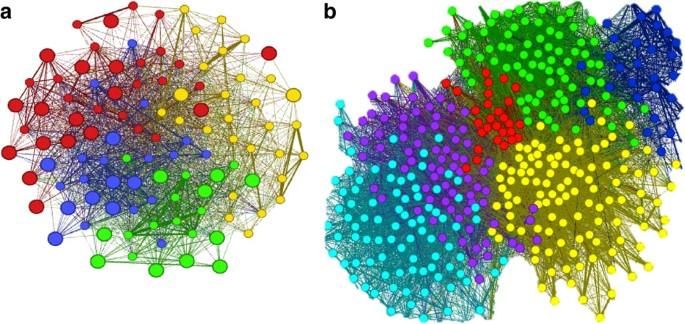Figure 3: Network clusters. (a) Shows four clusters for the 105 dolphins in the core sponger area. Larger nodes are spongers. Ties are weighted by the affinity index and represent clear cliques of spongers and non-spongers with a few interesting exceptions. The yellow cluster has 26 non-spongers and only 2 spongers, one old male and one old female (>30 years old). The red cluster has 18 non-spongers and 16 spongers, including 2 juvenile male spongers (<8 years old) that associate primarily with non-sponging males. The green cluster has ten spongers, all female, and ten non-spongers, all male members of one alliance (evident by tie strength). The blue cluster is virtually all male, with 5 male spongers, 15 non-sponging males and 3 young adult sponger females. (b) Shows six clusters for the entire network (439 dolphins). Spongers are in the purple and light blue clusters. All clusters correspond roughly to the areas these dolphins are sighted in. The red cluster is all-male with one exception. There were two main effects, one for sex (Wald test: z =−3.73, P <0.0001) and one for foraging type (Wald test: z =3.97, P <0.0001) and no significant interaction effects ( Table 3 ). Thus, males were less solitary than females and spongers were more solitary than non-spongers. Table 3 Parameter estimates and tests of fixed effects in GLMM of solitary and social surveys. Full size table Multiple Regression Quadratic Assignment Procedure We ran the MRQAP regression model in two ways, first including all dolphins within the core sponger area and second, by running males and females separately due to sex segregation in adult behaviour. Indeed, the negative MRQAP regression coefficient for matrilineal kinship in males countered the positive coefficient for matrilineal kinship in females. Statistical methods for directly testing for interactions with matrix data are still in development, and thus we were not able to explore the interaction of factors in this model. All explanatory variables predicted social affinity ( Table 4 ). Table 4 MRQAP regression model including males and females. Full size table The female only MRQAP model ( Table 5 ) showed results similar to those of the model including both sexes ( Table 4 ), although nearly twice the variance is explained. We excluded kinship from the Male MRQAP because there were too few pairs of maternally related dolphins. The Male MRQAP model continued to show that centroid location is a strong predictor of affinity (linear coefficient=−0.1391±0.0956, P =0.0140; log coefficient=−0.5647±0.0576, P =0.0005), but foraging homophily was not significant (sponger coefficient=0.01344±0.1128, P =0.2599; non-sponger coefficient=0.0532±0.1148, P =0.0565; 2,756 dyads; r 2 =0.196). Table 5 Female only MRQAP model. Full size table Community clusters We examined community clusters for dolphins in the core sponger area ( N =105, Fig. 3a ) and in the larger network ( N =439, Fig. 3b ) with the goal of finding groups with strong social affinity within a cluster and weaker social affinity outside the cluster. The spongers in Fig. 3a are the larger nodes and are concentrated in three of the four clusters. The spongers in the green cluster are all female and the majority of individuals in the red cluster are female (14 of 16). The blue cluster contains mostly males, both spongers and non-spongers (20 males and 3 females). Figure 3b shows six clusters for the entire community (439 dolphins). Spongers were grouped into two of the six clusters shown in Fig. 3b . Although spongers are clearly not a separate community or subcommunity and have many non-sponger associates in both figures, these clusters show that sponger homophily is imbedded in a larger subcommunity and spongers are not equally exposed to all subcommunities. Figure 3: Network clusters. ( a ) Shows four clusters for the 105 dolphins in the core sponger area. Larger nodes are spongers. Ties are weighted by the affinity index and represent clear cliques of spongers and non-spongers with a few interesting exceptions. The yellow cluster has 26 non-spongers and only 2 spongers, one old male and one old female (>30 years old). The red cluster has 18 non-spongers and 16 spongers, including 2 juvenile male spongers (<8 years old) that associate primarily with non-sponging males. The green cluster has ten spongers, all female, and ten non-spongers, all male members of one alliance (evident by tie strength). The blue cluster is virtually all male, with 5 male spongers, 15 non-sponging males and 3 young adult sponger females. ( b ) Shows six clusters for the entire network (439 dolphins). Spongers are in the purple and light blue clusters. All clusters correspond roughly to the areas these dolphins are sighted in. The red cluster is all-male with one exception. Full size image We set out to test whether sponge tool-use could be classified as cultural when culture is defined as both socially learned and distinguishes between groups. In dynamic fission–fusion societies lacking clear community boundaries, 'group' is better defined by relative affinity, as cliques or in terms of weighted (preferential) association. Spongers are imbedded in subcommunities and associate with non-spongers ( Fig. 3a,b ), but maintain strong homophily within their networks. In other animal societies, social preference based on tool-use or on socially learned traits per se has not been shown. Although in-group identity, based on socially learned traits, has been proposed for other species, such as group-specific calls in killer whales, Orcinus orca [33] , [34] and budgerigars, Melopsittacus-undulatus [35] , individuals within cultural subgroups exhibit similar calls as a consequence of affiliation. We suggest that spongers also share in-group identity, but affiliation is a consequence of similarity in the socially learned trait, a scenario that resonates with human culture [22] . Our results consistently supported the foraging homophily hypothesis for females, but not for males (discussed below). Spongers were more cliquish, had more sponger associates and stronger bonds with each other than with non-spongers. The significance of foraging homophily remained even after controlling for other factors that contribute to affiliation. These patterns are remarkable because spongers lead a relatively solitary lifestyle and have weaker ties with other dolphins than non-spongers do. Given that we included only non-spongers that are in the same habitat and had a very high chance of associating with spongers, our results are even more striking. The mutual interests of spongers seem to influence the nature of their social relationships. This is the first demonstration that a behaviour that is strictly vertically transmitted by a single parent serves an affiliative grouping function as well, thus meeting both criteria for culture. To date, no material subcultures have been identified outside of humans. While foraging type homophily held for females, it was weak for males. First, given the apparent social and geographic constraints of sponging, male spongers would have difficulty developing and maintaining effective alliances in their demographic. Only one male sponger dyad had an affinity index within the range of male alliances (>0.5 (ref. 31 )). Of the eight male spongers, five were in one cluster and are all young adults ( Fig. 3a ). The three other male spongers appeared to be split on age as well, with the single old male sponger in one cluster and the two youngest male spongers in another cluster. We know little about the circumstances that lead some males to sponge while others do not, but suspect that in addition to maternal influence, other associates have a role. Specifically, sons of spongers might use cues from their same-sex associates to determine whether sponging is a viable technique. For daughters, it might be more important to attend to maternal behaviour than their same sex cohort [36] . Once sponging behaviour is established, female spongers formed clear cliques ( Fig. 3a ) and were predominantly in two of four clusters ( Fig. 3a ). Interestingly, the exceptions were three female spongers that were in the otherwise all-male cluster ( Fig. 3a ). These females were young adults who have not successfully calved and were likely associating with males during repeated consortship events. All of the other sponger females were either juveniles or had successfully calved. Association patterns of these three spongers are likely to change once they have offspring. Despite extensive interaction between spongers and non-spongers, sponging does not spread horizontally or obliquely. According to the model proposed by Enquist et al . [37] , sponging would not represent shared cultural behaviour because vertically transmitted behaviours are not widely shared. That is, most vertically transmitted behaviours would not help in distinguishing between groups beyond kinship. Indeed, some hunting tactics in Shark Bay appear to be vertically transmitted, but are restricted to only a few individuals and might not involve preferential grouping outside of the matriline [14] , [28] . However, while spongers are a small minority of the population, the trait does help distinguish between groups or cliques and could thus qualify as cultural behaviour. Uniparental transmission does not necessarily preclude cultural behaviour. Homophily among spongers is likely to reinforce tool-use even though the calf has only one cultural parent. In a dynamic fission–fusion society, a variety of traits are likely to influence association, including sponging. In Shark Bay, tool-use with sponges is a lifestyle that impacts their activity budgets and social relationships. Shared lifestyles could also be a cue to relatedness, would enable more efficient information transfer and would reinforce sponging. As such, we do not exclude the possibility that horizontal transmission influences sponging behaviour (for example, prey patches, locations and types of sponges available) even though sponging is initially established through vertical transmission. Dolphins are substantial candidates for cultural behaviour given that they have a flexible social system, plastic behavioural repertoires, vocal learning abilities, a high social tolerance, slow life histories, imitation abilities and large brains [29] , [38] , [39] , [40] , [41] . We do not argue that foraging type is the primary determinant of association. Dolphin association is likely to be driven by multiple factors, including a suite of contexts such as behavioural state [42] , foraging type, the history of interactions, reproductive state, and enduring traits such as sex [25] , [26] , [31] , kinship [30] , [43] , age [44] and geography [30] . Homophily on a variety of traits has a critical role in human (sub)cultures [22] and this may be true for dolphin society as well. Sponging is unlikely to be the only socially learned behaviour related to the frequency of association. Calves tend to be socially similar to their mothers, suggesting that social network patterns might be socially transmitted [36] . Adult males appear to converge on signature whistles within an alliance over time [45] , [46] , suggesting that there are affiliative functions to other socially learned behaviours. These are instances where affiliation drives the socially learned trait, rather than the reverse. Cultural processes are integral to evolutionary dynamics. Under certain conditions, selection is expected to favor social learning mechanisms and biases; the resulting behaviours are then favoured by socio-ecological and other processes, thereby reinforcing the evolution of social learning. In the dynamic, inherently flexible fission–fusion social system that Shark Bay bottlenose dolphins live in, individuals vary on a wide range of features: sociability, network structure, alliance formation, life history traits, habitat use and foraging tactics [10] , [11] , [14] , [21] , [25] , [26] , [29] , [31] , [36] . Social tolerance, at least between females [38] , and low travel costs [47] allow dolphins from different cliques and subcommunities to associate with each other, including those with distinct attributes, histories and lifestyles. The challenges of these diverse encounters might have shaped the evolution of individual variation, innovation, cognition and plasticity in dolphin populations, all of which contribute to the evolution of cultural behaviour. Study site Our main study site encompasses ∼ 300 km 2 in the eastern gulf of Shark Bay, Western Australia (25°47′S 113°43′E). Over 1,500 residential bottlenose dolphins ( Tursiops sp.) have been surveyed since 1984. Surveys Surveys are opportunistic sightings of dolphins where the presence of individuals during a 5-min interval is recorded. Dolphins were identified by photo-ID (distinctive body and dorsal fin markings). Association was determined via a 10-m chain rule, in which individuals were considered to be associated if they were within 10 m of each other or similarly linked by another. Behavioural, demographic, reproductive and ecological data were also recorded. The current study used 14,651 surveys collected annually from 1989 to 2010. Data restrictions The survey sample included all dolphins with >11 sighting records across 3 or more years post-weaning (average±s.e. surveys per dolphin, 99.5±6.3; N =439, 212 females, 209 males). Dependent calves were excluded from all analyses. To limit the sample to animals with which spongers would have the greatest possibility of associating with and who experience the same ecological context as spongers, we calculated centroids for all 439 dolphins and further restricted our sample to animals that fell within a minimum convex polygon (MCP) created around the 36 sponger centroids in this sample ( Fig. 2 ). A centroid corresponds to an average latitude and longitude and is a good measure of the central tendency of an animal's location [48] . Only the last location point was used per day for each dolphin to reduce biases associated with our boat-launching site. The sponger MCP ( Fig. 2 ) includes 105 dolphins (53 males, 52 females; 74.7±5.5 surveys per dolphin) that are most likely to encounter spongers based on location and experience the same habitat as spongers. All but one of the 105 dolphins associated with a sponger at least once. That is, we intentionally restricted our analysis to a sample that would be least likely to support the homophily hypothesis, because spongers and non-spongers would have a very high chance of association based on geographic location alone. Dolphin home ranges are typically more than twice the size of the sponger MCP [27] . We deliberately chose a smaller area so that there was complete geographic overlap between spongers and non-spongers. Finally, because spongers are more solitary than non-spongers [10] , we analysed the data by first including all survey records, and second, by excluding all solitary sightings for a dolphin. Because the results were identical, we report results that used all sighting data. Social metrics Owing to demographic changes, some dolphins were sighted over the entire 22-year period, while others were sighted for a subset. Thus, we chose the social affinity index because it generally excludes demographic effects [49] . Social affinity indices were calculated in SOCPROG 2.4 (2010) using the following formula: x /Min{( x + y AB + y A ),( x + y AB + y B )}, where x is the number of sampling days that A and B were observed together; y A is the number of sampling days that A was observed without B, y B is the number of sampling days that B was observed without A and y AB is the number of sampling days in which A and B were both observed, but not together. We also directly accounted for the complete lack of temporal overlap between some dolphins (for example, a grandmother dies before her granddaughter is born) by coding data as missing for a given dyad if they did not overlap. All network ties were weighted based on the social affinity matrix. Weighting or quantifying the strength of ties is particularly critical in fission–fusion societies, where the frequency with which individuals are observed together is important to capture. We examined foraging type and sex differences for five major social network metrics: degree, strength, betweenness, eigenvector centrality and clustering coefficient. Degree is the number of nodes (associates) that an individual is directly connected to (that is, total number of individual dolphins that a dolphin was sighted with). Strength, also known as weighted degree, is the sum of weighted ties (social affinity indices for these analyses) for a given individual. Betweenness is a measure of how often an individual falls on the shortest path connecting other individuals in the network. Eigenvector centrality is a measure of an individual's importance in the network and is determined as the distance from other central individuals relative to all others in the network. Clustering coefficient is a measure of cliquishness or how likely it is that the associates of one individual are also directly connected to each other. Non-social metrics Non-social variables included sex, foraging type, kinship and location. We documented matrilineal relatedness for 28 of 36 spongers (known mother and/or offspring, including some offspring that did not adopt sponging) and for 98 of non-spongers; genetic relatedness was known for only 14 of these spongers [13] , [15] . As we have documented matrilineal relationships for 27 years, these data represent kinship that dolphins themselves would recognize through association with the mother, although additional kin recognition mechanisms are possible [30] . Centroid distances (km) between each dyad were calculated as a measure of geographic proximity. Analyses We examined differences in basic social network metrics between males and females as well as between spongers and non-spongers using two-sample permutation tests (R v.2.13.0, 10,000 permutations) with all confidence intervals >0.99. Because male social metrics differ from females ( Table 1 ) and most spongers are female, we restricted some of our comparisons to females only. To determine whether there was a difference between sponger and non-sponger within versus between-group associations, we used a Mantel test to test for a correlation between matrices. A Mantel test generates a test statistic quantifying the association between two matrices, and then permutes them to generate a null distribution for the test statistic, allowing us to calculate a P -value quantifying the strength of evidence against the null hypothesis of no underlying association. We used a generalized linear mixed model with binomial error structures and logit link function to examine sociability (# of sightings alone versus not alone) with sex, foraging type and their interaction as fixed effects, and individual as a random effect. To test whether similarity in maternal kinship, foraging type (sponger and non-sponger) sex and/or geographic proximity were significant predictors of associations, we used the Double Dekker Semi-Partialling MRQAP [32] in UCINET 6 (ref. 50 ). QAP regression is a type of Mantel test that allows for a response matrix to be regressed against multiple explanatory matrices that represent dyadic attribute relationships. QAP first runs a standard OLS regression and then randomly permutes the rows and columns of the dependent matrix (2,000× here), recalculating the regression and creating a matrix-specific distribution against which the R 2 and coefficients of the observed matrix can be compared to determine significance. Thus, MRQAP regression examines and controls for multiple factors when parameterizing a continuous dependent variable, and the results can be interpreted similar to those of standard multiple regression; however, the permutation approach accounts for the structural autocorrelation inherent to social network data [32] . Note that due to the limit on the number of possible correlations imposed by the structure of network data, the R 2 of QAP regression is smaller than in OLS regression [32] , [51] . Social affinity indices were the response matrix, while maternal relatedness, distance between centroids (geographic proximity), log transformed distance between centroids, sex homophily and foraging type homophily (sponger and non-sponger) served as explanatory matrices. Sex homophily matrices were created by assigning a value of 1, if two dolphins were the same sex, and 0 otherwise. Two foraging type matrices were created; one in which sponger similarity was assigned a value 1, and one in which non-sponger similarity was assigned a value of 1. Dissimilar dyads were coded as 0. Separate sponger and non-sponger homophily matrices allowed us to determine whether similarity between one, both or neither groups contributed to association. To examine the position of spongers within the larger population, we applied a community detection algorithm to our social affinity matrices. The goal of such algorithms is to find clusters with strong connectivity and group them together. While a number of different algorithms exist, we used one which uses spin glass quality function from magnetic systems and modularity optimization in its computation [52] . How to cite this article: Mann, J. et al . Social networks reveal cultural behaviour in tool-using using dolphins. Nat. Commun. 3:980 doi: 10.1038/ncomms1983 (2012).